Expansion of host cellular niche can drive adaptation of a zoonotic malaria parasite to humans The macaque malaria parasite Plasmodium knowlesi has recently emerged as an important zoonosis in Southeast Asia. Infections are typically mild but can cause severe disease, achieving parasite densities similar to fatal Plasmodium falciparum infections. Here we show that a primate-adapted P. knowlesi parasite proliferates poorly in human blood due to a strong preference for young red blood cells (RBCs). We establish a continuous in vitro culture system by using human blood enriched for young cells. Mathematical modelling predicts that parasite adaptation for invasion of older RBCs is a likely mechanism leading to high parasite densities in clinical infections. Consistent with this model, we find that P. knowlesi can adapt to invade a wider age range of RBCs, resulting in proliferation in normal human blood. Such cellular niche expansion may increase pathogenesis in humans and will be a key feature to monitor as P. knowlesi emerges in human populations. Cross-species transmission of malaria parasites is extremely rare, with host-specific vectors and molecular barriers to infection maintaining species boundaries. The intensification of human activities such as farming and logging, however, have led to the emergence of zoonotic infections with the macaque malaria parasite Plasmodium knowlesi among human populations in Southeast Asia [1] , [2] , [3] , [4] . Currently, most P. knowlesi- infected humans experience extremely low parasite densities in the blood, presumably due to the parasite’s inability to replicate efficiently in human red blood cells (RBCs), and this is one of the reasons there is no continuous in vitro culture system (the equivalent of batch culture for bacteria) in human blood. Increasingly, however, individuals suffer severe disease associated with greater than 20-fold increases in parasite densities, comparable with highly virulent Plasmodium falciparum infections [5] , [6] , [7] . These high parasitaemia infections raise the concern that parasite adaptations increasing proliferation in human hosts may dramatically increase the virulence of clinical infections. Human RBCs undergo substantial morphological and functional change during their 4-month lifespan, and represent a dynamic and heterogeneous population of potential target cells for malaria parasite invasion [8] . Several Plasmodium species show preferences for limited subpopulations of circulating RBCs and these restrictions may constrain peak parasite density in vivo , a key predictor of disease outcome. Of the four human malaria parasites, P. vivax [9] and P. ovale [10] are restricted to the youngest RBCs called reticulocytes and P. malariae to older normocytes [11] . Only the highly virulent P. falciparum is able to efficiently invade RBCs of all ages [12] , [13] . It is thought that this broader host cellular niche underlies the ~10-fold higher parasite densities observed for P. falciparum compared with the other human malaria parasites [6] , [7] , [10] , [14] . P. knowlesi can invade both reticulocytes and normocytes in its natural host, the long-tailed macaque [15] , as well as in the rhesus macaque animal model [16] . However, its ability to invade different subsets of human RBCs and the extent to which RBC age heterogeneity affects the proliferation of P. knowlesi during zoonotic infections is unknown. Here we show that the heterogeneity of RBC age in normal human blood restricts the proliferation of P. knowlesi . We establish a continuous in vitro culture system in human RBCs by enriching with particular RBC subsets, yielding a powerful and readily accessible system for further experimental investigation. Using a mathematical model, we predict that parasite adaptations allowing for the invasion of a broad age range of RBCs will increase in vivo peak parasite densities more efficiently than the enhancement of intrinsic growth rates. We then demonstrate that a primate-adapted P. knowlesi strain can dramatically expand its age range of target cells following prolonged culture in human RBCs, providing a second in vitro culture system. This type of adaptation for proliferation in human hosts may significantly increase pathogenesis [17] , [18] , [19] . P. knowlesi is restricted to young human RBCs To investigate the effect of host cell age on P. knowlesi invasion of human RBCs, we compared the invasion ability of the P. knowlesi H strain to that of the P. falciparum lab strain 3D7 in human RBCs of varying age. This P. knowlesi strain was originally isolated from a human traveller returning from Malaysia in 1965, most likely from a zoonotic infection, and has since been passaged through rhesus macaque monkeys and subsequently adapted in vitro in rhesus macaque RBCs [3] , [20] . For both this strain and the 3D7 lab strain, we measured the fold change in parasitaemia following a single round of invasion (the ‘Parasitized Erythrocyte Multiplication Rate’ or PEMR [13] ) into ‘very young’, ‘young’, ‘medium’ and ‘old’ age fractions of human RBCs, as well as a control of pooled blood fractions (see Methods and Fig. 1a–c ) [21] , [22] . As expected, the PEMR was much lower for the P. knowlesi strain into the human pooled blood fraction compared with the P. falciparum strain ( Fig. 1d ). Strikingly, P. knowlesi exhibited a dramatic decrease in invasion into progressively older RBC fractions, accounting for its low invasion potential overall. In contrast, P. falciparum only showed a slight decline in invasion efficiency into older RBC fractions, as previously described [12] . The skew in age preference between the two parasites is contrasted in Fig. 1e , which measures the invasion efficiency into different age fractions relative to the pooled control for both species. 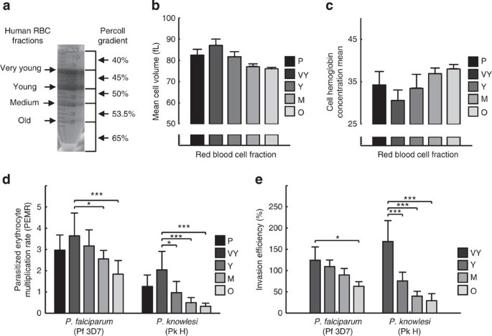Figure 1:P. knowlesiH strain invades young human red blood cells more efficiently. (a) The density of red blood cells increases with age as their volume decreases, attributable to loss of plasma membrane and cytoplasm without concomitant expulsion of intracellular contents such as haemoglobin. They can thus be separated into four fractions by layering them on top of an optimized gradient of Percoll solutions. This is validated by measuring (b) mean cell volume (MCV) and (c) cell haemoglobin concentration mean (CHCM). MCV decreases in the older subpopulations of red blood cells while CHCM increases. Ninety-five per cent confidence interval (CI) for three replicates are shown. (d) Fold change in parasitemia following a single round of invasion, the PEMR, forP. falciparum3D7 andP. knowlesiH strain into human red blood cell populations of varying age fractions, measured in parallel. (e) Skew in age preference measured as the normalized invasion efficiency ofP. falciparum3D7 andP. knowlesiH strain in each age category relative to the pooled control for each species. Data are from six biological replicates. Statistical significance was determined using a two-way analysis of variance with a Bonferroni correction for multiple comparisons. Ninety-five per cent CI are shown; *P<0.05; **P<0.01; ***P<0.001; P, pooled blood; VY, very young red blood cells; Y, young red blood cells; M, medium age red blood cells; O, old red blood cells. Figure 1: P. knowlesi H strain invades young human red blood cells more efficiently. ( a ) The density of red blood cells increases with age as their volume decreases, attributable to loss of plasma membrane and cytoplasm without concomitant expulsion of intracellular contents such as haemoglobin. They can thus be separated into four fractions by layering them on top of an optimized gradient of Percoll solutions. This is validated by measuring ( b ) mean cell volume (MCV) and ( c ) cell haemoglobin concentration mean (CHCM). MCV decreases in the older subpopulations of red blood cells while CHCM increases. Ninety-five per cent confidence interval (CI) for three replicates are shown. ( d ) Fold change in parasitemia following a single round of invasion, the PEMR, for P. falciparum 3D7 and P. knowlesi H strain into human red blood cell populations of varying age fractions, measured in parallel. ( e ) Skew in age preference measured as the normalized invasion efficiency of P. falciparum 3D7 and P. knowlesi H strain in each age category relative to the pooled control for each species. Data are from six biological replicates. Statistical significance was determined using a two-way analysis of variance with a Bonferroni correction for multiple comparisons. Ninety-five per cent CI are shown; * P <0.05; ** P <0.01; *** P <0.001; P, pooled blood; VY, very young red blood cells; Y, young red blood cells; M, medium age red blood cells; O, old red blood cells. Full size image P. knowlesi culture in human blood enriched with young cells P. falciparum is the only human malaria parasite for which a robust in vitro culture system in human blood is available [23] . On the basis of the preference for young RBCs we observed for P. knowlesi H, we hypothesized that an artificial enrichment of young RBCs may allow for the establishment of a continuous in vitro culture system for P. knowlesi in human blood. Cultures of P. knowlesi H with different proportions of very young RBCs were initiated (see Methods). As the proportion of very young RBCs increased, measured as the percentage of reticulocytes, the PEMR of the P. knowlesi H strain rose dramatically ( Fig. 2a ). To assess the ability of parasites to proliferate within these age fractions, cultures were grown in parallel in a continuous culture system (see Methods). In non-enriched human blood, the parasite quickly died out ( Fig. 2b ), but as the proportion of young cells increased, the parasite was able to sustain successive rounds of replication. Continuous culture was successfully established in blood enriched with >8% reticulocytes, and was maintained continuously for 6 months. These results confirm that RBC age heterogeneity restricts the proliferation of P. knowlesi parasites and also provide for the first time a continuous culture system in human blood for future experimental investigations of the P. knowlesi parasite biology in human RBCs. 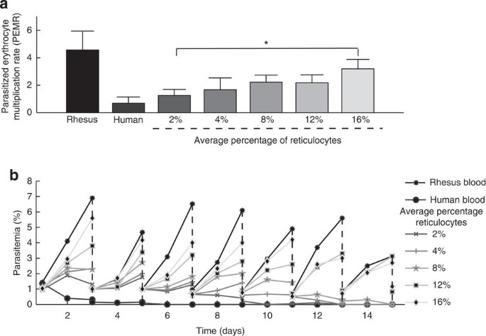Figure 2: Continuousin vitroculture established by increasing the number of young red blood cells. (a) PEMR ofP. knowlesiH strain in cultures with different proportions of very young red blood cells after one round of reinvasion, as calculated in Figure 1. Statistical significance was determined using Dunnett’s multiple comparison test. Ninety-five per cent confidence interval for five replicates are shown; *P<0.05. (b) Parasitemia ofP. knowlesiH strain in cultures with different proportions of very young red blood cells, compared with rhesus blood (small circles), and human blood (large circles). H was continuously cultured in the different proportions by sub-culturing them every 2 days (dashed lines) and parasitemia monitored daily, before and after the split. Figure 2: Continuous in vitro culture established by increasing the number of young red blood cells. ( a ) PEMR of P. knowlesi H strain in cultures with different proportions of very young red blood cells after one round of reinvasion, as calculated in Figure 1. Statistical significance was determined using Dunnett’s multiple comparison test. Ninety-five per cent confidence interval for five replicates are shown; * P <0.05. ( b ) Parasitemia of P. knowlesi H strain in cultures with different proportions of very young red blood cells, compared with rhesus blood (small circles), and human blood (large circles). H was continuously cultured in the different proportions by sub-culturing them every 2 days (dashed lines) and parasitemia monitored daily, before and after the split. Full size image RBC age preference restricts in vivo parasitaemia Among human and rodent malaria parasite species, RBC age preferences have been linked to broad differences in peak parasite densities and resulting pathogenesis [24] , [25] , [26] , [27] . We used a mathematical model of RBC ageing and the 24-h asexual lifecycle of P. knowlesi infections (see Methods, Equations (1) and (3)) to evaluate three possible mechanisms that could account for the dramatically increased peak parasite densities observed in a few human P. knowlesi infections. Specifically, we compared the effects of (i) increasing the intrinsic invasion ability β (a measure of the intrinsic ability of a merozoite to invade a susceptible cell, see Methods, Equation (1)) within the current niche of very young RBCs, (ii) increasing the number of susceptible host cells by increasing the proportion of very young cells, as would occur in anaemic hosts and (iii) shifting the parasite’s cellular niche by increasing the susceptible age range to include older cells ( Fig. 3 ). Owing to its low prevalence in humans, most P. knowlesi parasites are unlikely to encounter hosts with adaptive immune responses, and we focus on initial parasite replication in the absence of an immune response like previous frameworks [24] , [27] . 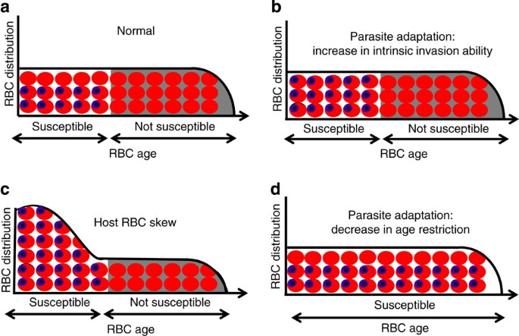Figure 3: Potential mechanisms leading to increased parasite proliferation. Schematics show the density of red blood cells (vertical axis) as they age (horizontal axis), with infected cells containing parasites (in blue). (a) At baseline,P. knowlesihas a limited intrinsic invasion abilityβand an invasion niche restricted to young red blood cells. Increased parasite proliferation can be achieved by (b) increasing the parasite’s intrinsic invasion ability within this niche, (c) skewing the distribution of red blood cells in the host to increase the proportion of young cells or (d) expanding the parasite’s invasion niche to include older cells. Figure 3: Potential mechanisms leading to increased parasite proliferation. Schematics show the density of red blood cells (vertical axis) as they age (horizontal axis), with infected cells containing parasites (in blue). ( a ) At baseline, P. knowlesi has a limited intrinsic invasion ability β and an invasion niche restricted to young red blood cells. Increased parasite proliferation can be achieved by ( b ) increasing the parasite’s intrinsic invasion ability within this niche, ( c ) skewing the distribution of red blood cells in the host to increase the proportion of young cells or ( d ) expanding the parasite’s invasion niche to include older cells. Full size image The model suggests that increasing the fraction of susceptible cells, either through parasite adaptation or a skewed RBC distribution, has a much greater impact on peak parasite density than simply enhancing the parasite’s intrinsic invasion ability β ( Fig. 4a ). This is because the effective reproduction number R e (see Equation (2)) is approximately proportional to the density of susceptible cells ( Fig. 4b ) consistent with mouse models [28] , [29] . We find that the highly skewed distribution of RBCs required to attain high parasite densities, analogous to the in vitro culture system described above, would be associated with severe anaemia ( Fig. 5 ), and this has not been observed in P. knowlesi infections [5] , [7] , [30] . We therefore predict that parasite adaptation to invade a wider range of RBC ages can plausibly explain the large increases in parasite density observed in clinical P. knowlesi cases. 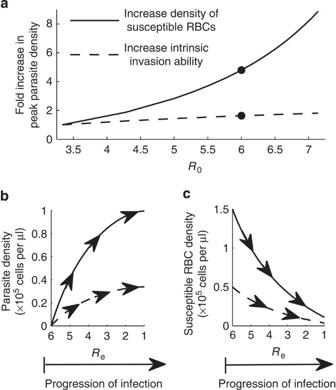Figure 4: Comparison of different adaptive pathways on predictedin vivopeak parasite densities. (a) Relative changes in peak parasite density (initialR0=3.3 and the parasite can invade red blood cells during the first 20% of their lifespan). IncreasingR0from this baseline is achieved either by increasing the intrinsic invasion abilityβof susceptible cells (dashed line) or by increasing the age range of red blood cells that are susceptible to invasion (solid line) up to 100%. (b) Parasite density as the infection progresses for parasites that have attained anR0=6 by either increasing the density of susceptible cells (corresponding to point on solid curve in Fig. 3a), or by increasing their intrinsic invasion abilityβ(corresponding to point on dashed curve in Fig. 3a). The peak parasite density occurs when Re=1 and is higher for the parasite with an increased density of susceptible cells (solid curve) than for the parasite with increased intrinsic invasion abilityβ(dashed curve). (c) Changes in susceptible cell density for infection dynamics in Fig. 3b. As infection progresses, the density of susceptible cells declines. The net decrease in susceptible cell density due to invasion is much greater for the parasite with a higher initial density of susceptible RBCs (solid curve) than for the parasite with increased intrinsic growth (dashed curve). Figure 4: Comparison of different adaptive pathways on predicted in vivo peak parasite densities. ( a ) Relative changes in peak parasite density (initial R 0 =3.3 and the parasite can invade red blood cells during the first 20% of their lifespan). Increasing R 0 from this baseline is achieved either by increasing the intrinsic invasion ability β of susceptible cells (dashed line) or by increasing the age range of red blood cells that are susceptible to invasion (solid line) up to 100%. ( b ) Parasite density as the infection progresses for parasites that have attained an R 0 =6 by either increasing the density of susceptible cells (corresponding to point on solid curve in Fig. 3a), or by increasing their intrinsic invasion ability β (corresponding to point on dashed curve in Fig. 3a). The peak parasite density occurs when R e =1 and is higher for the parasite with an increased density of susceptible cells (solid curve) than for the parasite with increased intrinsic invasion ability β (dashed curve). ( c ) Changes in susceptible cell density for infection dynamics in Fig. 3b. As infection progresses, the density of susceptible cells declines. The net decrease in susceptible cell density due to invasion is much greater for the parasite with a higher initial density of susceptible RBCs (solid curve) than for the parasite with increased intrinsic growth (dashed curve). 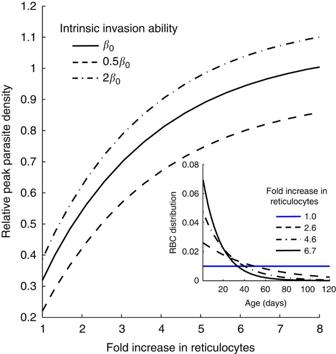Figure 5: Relative peak parasite densities for hosts with skewed red blood cell age distributions. Each curve shows the peak parasite density for a parasite restricted to very young cells, but invading hosts with different red blood cell age distributions (as distinguished by the fold increase in reticulocytes compared to a healthy host). All peak parasite densities are relative to the peak parasite density attained by a parasite that can invade cells of all ages in a healthy host and baseline intrinsic invasion ability (β0). Each curve represents a different intrinsic invasion ability for the restricted parasite:β0(solid), 0.5β0(dashed), 2β0(dot-dashed). The baseline intrinsic invasion abilityβ0was chosen so that in a healthy host, a parasite restricted to very young cells has aR0=5. Inset shows examples of different host red blood cell age distributions. A skewed host distribution is modelled by assuming that an elevated rate of RBC destruction across all cell ages is compensated for by an increased production of reticulocytes. It is assumed that the increased production of reticulocytes is sufficient to maintain a normal density of RBCs (5 million cells per μl). The fold increase in reticulocytes for the skewed distributions (inset: black curves) is calculated relative to the RBC distribution of a normal host (inset: blue curve). Full size image Figure 5: Relative peak parasite densities for hosts with skewed red blood cell age distributions. Each curve shows the peak parasite density for a parasite restricted to very young cells, but invading hosts with different red blood cell age distributions (as distinguished by the fold increase in reticulocytes compared to a healthy host). All peak parasite densities are relative to the peak parasite density attained by a parasite that can invade cells of all ages in a healthy host and baseline intrinsic invasion ability ( β 0 ). Each curve represents a different intrinsic invasion ability for the restricted parasite: β 0 (solid), 0.5 β 0 (dashed), 2 β 0 (dot-dashed). The baseline intrinsic invasion ability β 0 was chosen so that in a healthy host, a parasite restricted to very young cells has a R 0 =5. Inset shows examples of different host red blood cell age distributions. A skewed host distribution is modelled by assuming that an elevated rate of RBC destruction across all cell ages is compensated for by an increased production of reticulocytes. It is assumed that the increased production of reticulocytes is sufficient to maintain a normal density of RBCs (5 million cells per μl). The fold increase in reticulocytes for the skewed distributions (inset: black curves) is calculated relative to the RBC distribution of a normal host (inset: blue curve). Full size image P. knowlesi can adapt to invade RBCs of all ages We next tested whether P . knowlesi parasites are able to increase their within-host basic reproduction number in humans and adapt to proliferate in normal, un-enriched human blood. P. knowlesi H strain was first cultured in vitro on a mixture of rhesus and human RBCs (10:90) for a month, then shifted for growth on human RBCs (100%). After 4 months, a parasite line (H hu ) was able to proliferate at a stable rate in normal human blood ( Fig. 6a ). When the invasion of this adapted parasite into RBCs of different age was measured, the striking age preference for young RBCs observed in the primate-adapted P. knowlesi H strain was greatly altered, and overall PEMR was substantially increased as a result ( Fig. 6b ). The adapted strain H hu was able to efficiently invade all age groups of human RBCs ( Fig. 6c ), in a pattern similar to the P. falciparum parasite ( Fig. 1d ). 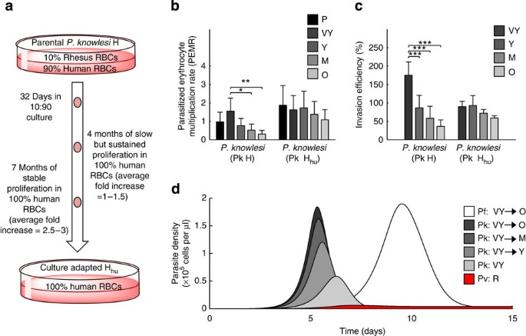Figure 6:P. knowlesiH strain adapts to proliferate in normal human blood. (a) Schematic timeline for production of aP. knowlesiline (Hhu) adapted toin vitroculture in normal human red blood cells. (b) PEMR of primate-adaptedP. knowlesiH strain compared with the human-adapted strainP. knowlesiHhuinto human red blood cell populations of varying age, and (c) relative invasion efficiency ofP. knowlesiH and Hhuinto red blood cell populations of varying age, calculated as in Fig. 1. Ninety-five per cent confidence interval for five biological replicates are shown. Statistical significance was determined using a two-way analysis of variance analysis with a Bonferroni correction for multiple comparisons. *P<0.05; **P<0.01; ***P<0.001. (d) Predictedin vivoinfection dynamics assuming an approximately uniform distribution of RBCs for (i)P. vivax(Pv) restricted to reticulocytes (R) (red), (ii)P. falciparum(Pf) able to invade red blood cells of all ages (white), (iii)P. knowlesi(Pk) restricted to very young (VY) red blood cells (very light grey), (iv) Pk restricted to very young and young (VYY) red blood cells (light grey), (v) Pk able to invade very young to medium (VYM) red blood cells (medium grey) and (vi) Pk able to invade red blood cells of all ages (VYO) (dark grey). For ease of interpretation, we assume that (i) the initial parasite invasion rates for Pv, Pf and the Pk strain restricted to very young cells are the same and (ii) the intrinsic invasion abilities of all Pk strains are the same. Figure 6: P. knowlesi H strain adapts to proliferate in normal human blood. ( a ) Schematic timeline for production of a P. knowlesi line (H hu ) adapted to in vitro culture in normal human red blood cells. ( b ) PEMR of primate-adapted P. knowlesi H strain compared with the human-adapted strain P. knowlesi H hu into human red blood cell populations of varying age, and ( c ) relative invasion efficiency of P. knowlesi H and H hu into red blood cell populations of varying age, calculated as in Fig. 1. Ninety-five per cent confidence interval for five biological replicates are shown. Statistical significance was determined using a two-way analysis of variance analysis with a Bonferroni correction for multiple comparisons. * P <0.05; ** P <0.01; *** P <0.001. ( d ) Predicted in vivo infection dynamics assuming an approximately uniform distribution of RBCs for (i) P. vivax (Pv) restricted to reticulocytes (R) (red), (ii) P. falciparum (Pf) able to invade red blood cells of all ages (white), (iii) P. knowlesi (Pk) restricted to very young (VY) red blood cells (very light grey), (iv) Pk restricted to very young and young (VY Y) red blood cells (light grey), (v) Pk able to invade very young to medium (VY M) red blood cells (medium grey) and (vi) Pk able to invade red blood cells of all ages (VY O) (dark grey). For ease of interpretation, we assume that (i) the initial parasite invasion rates for Pv, Pf and the Pk strain restricted to very young cells are the same and (ii) the intrinsic invasion abilities of all Pk strains are the same. Full size image Using the mathematical model, we compared the peak parasite densities expected in vivo for parasite species with equivalent parasite invasion rates (see Methods) but different RBC age preferences and lengths of asexual RBC cycles. Figure 6d shows the peak parasitaemia for a P. knowlesi parasite with different age preferences relative to analogous peaks for P. falciparum and P. vivax parasites under the assumption that the maximum possible level of parasitaemia is 5% (see Methods). We envisage that these scenarios represent the potential dynamics of a human-adapted P. knowlesi parasite. In this case, the peak parasite density of the P. knowlesi parasite with no pronounced age preference is similar to that of a P. falciparum parasite. Compared with P. falciparum , however, P. knowlesi ’s shorter RBC cycle causes its parasite density to peak earlier, and its lower number of daughter parasites (merozoites) per cell leads to a lower cumulative parasite density. Given the potential for this P. knowlesi strain to expand its cellular niche to include older RBCs, our results suggest that this type of parasite adaptation in field isolates may lead to dramatic increases in parasite density in vivo . RBCs represent a dynamic and heterogeneous landscape for invasion of malaria parasites. Here, we show that the limited proliferation of P. knowlesi H parasite observed in human RBCs is due to its marked preference for the youngest subpopulation of cells. We have developed two distinct systems for the continuous in vitro culture of P. knowlesi . First, providing the parasite with large numbers of very young RBCs can greatly enhance the proliferative potential of this P. knowlesi parasite, leading to its propagation in human blood. This may readily allow for the culture adaptation of P. knowlesi from both human infections and from macaque hosts. Enriched cells can also be used in the development of field deployable assays to study phenotypes such as inhibition of RBC invasion and drug susceptibility. Our second culture system, the normocyte-adapted parasite line can lead to P. knowlesi proliferation in normal human blood using standard culture conditions. Together, these culture systems will enable further investigation of P. knowlesi biology without the requirement for primate facilities, allowing for the dissemination to multiple laboratories. P. knowlesi will be particularly useful as a model system for cell biological studies, due to the relatively large size and stability of the invasive merozoite form [31] , [32] , and will provide a powerful system for genetic analyses [33] . It also provides a relevant in vitro model for the evolutionarily related P. vivax malaria parasite, which currently lacks an in vitro culture system, as well as facilitates the exploration of numerous questions of comparative biology of malaria parasites. Indeed, the principles that we have established may help to establish P. vivax in vitro culture. Coevolution between humans and malaria parasites has led to a range of human genetic polymorphisms encoding RBC heterogeneity on a population level [34] . These mutations may restrict parasite proliferation in vivo , as exemplified by the reduced parasite densities and disease severity afforded by the sickle cell trait [35] , [36] , and the selection against the DARC surface receptor, which is required for P. vivax invasion, in large areas of sub-Saharan Africa [37] , [38] . Differences between host species in RBC surface receptors required for invasion are also likely to be a major barrier for zoonotic transmission of malaria parasites between species [39] . Here, however, we have demonstrated that in addition to genetic variation within and between species, RBC heterogeneity resulting from the ageing process within individuals represents another significant level of restriction to the evolution of a zoonotic infection. It is likely that the shift in age preference exhibited by our adapted line is linked to changes in the utilization of P. knowlesi invasion ligands, as has been observed in rodent malaria parasites [40] . Interestingly, the considerable length of time required for our human-adapted line to emerge suggests that the underlying changes were of genetic rather than epigenetic origin. Identifying these changes and determining their relevance in human isolates will be an important next step. We propose that de novo P. knowlesi adaptation allowing invasion of older cells may be an important driver of the high parasite densities observed in severe clinical P. knowlesi cases. Although the host and parasite mechanisms underlying clinical malaria are complex, high parasite densities have consistently been found to be most strongly associated with severe disease among P. knowlesi infections in the field [5] , [6] , [7] . The analyses presented here focus on single species infections, but coinfection with other human malaria parasites is relatively common for P. knowlesi infections [41] , [42] and could also impact the severity of infection [43] , as could other underlying conditions causing anaemia. Interestingly, increased parasite densities in vivo would also increase the effective parasite population size, enhancing the likelihood of the emergence of transmissible parasites in humans. Previous theoretical work has shown that only modest between-host R 0 values are required for the spread and maintenance of emerging pathogens in human populations if pathogen mutability is high [19] . However, transmission between humans is likely to rely on a range of complex and poorly understood parasite and vector-related factors, such as the production of viable parasite transmission stages and the availability of anthropogenic vectors. Although human infections are still limited in their geographical range by vector distributions [44] , [45] , the continuing encroachment of human populations on macaque habitat provides increasing exposure to non-human primate malaria parasites. Strikingly, although humans are likely to be frequently exposed to numerous related cynomolgous malaria parasites, such as P. cynomolgi and P. inui , P. knowlesi is unique in its emergence into human populations [2] , [46] . Here we have elucidated one of the host factors currently limiting its proliferation in human blood, and highlighted the intrinsic capacity of the parasite to increase its invasion potential by adapting to heterogeneous host RBCs. We propose that this mechanism of expansion of RBC age preferences of P. knowlesi field strains will be a critical feature to monitor as zoonotic P. knowlesi infections increase. Of concern, parasites that are more virulent were readily obtained following continuous in vivo passage of P. knowlesi in humans for the treatment of neurosyphilis [47] . Parasite culture P. knowlesi H was provided by Dr. A. Thomas (Biomedical Primate Research Center, Rijswijk). P. falciparum 3D7 was from the Walter and Eliza Hall Institute (Melbourne, Australia). Parasites were maintained in vitro in rhesus ( P. knowlesi ) or human 0+ RBCs ( P. falciparum ) at 2% haematocrit using standard culture conditions [20] , [23] . Parasitemia was determined by light microscopy. Density-dependent separation of human RBCs Uninfected human RBCs were incubated at 37 ° C for 30 h and separated by density into distinct subpopulations of different age. Five Percoll solutions of increasing concentration (40%, 45%, 50%, 53.5% and 65% in RPMI) were overlaid into a 15-ml falcon tube, 2 ml each, beginning with the densest solution [21] , [22] . Six hundred microlitre of human RBCs at 30% haematocrit that had been incubated for 30 h were added on top of the layer, and centrifuged (1,200 g /12 mins). Each cell layer was collected and washed. Mean cell volume and the cell haemoglobin concentration mean of each fraction were determined on an ADVIA haematological analyser (Bayer) ( Fig. 1a–c ). Measuring invasion into RBCs. Magnet-purified schizonts (95% purity) were added at a parasitaemia of 0.7–1% to 150 μl cultures at 2% haematocrit of age-fractionated RBCs, and incubated at 37 ° C for reinvasion. As a control, the fractionated sup-populations were repooled according to the average volume of RBCs obtained after the process (on average, 40% of the RBCs were found in very young fraction, 30% in young, 20% in medium and 10% in the oldest fraction). This control was thus representative of the whole blood, yet subjected to the same manipulations. The PEMR was determined by dividing the final parasitaemia at rings by the initial parasitaemia of schizonts [13] . Invasion efficiency was determined as the ratio of the PEMR of the parasite strain in each blood fraction to the PEMR in the pooled fraction, converted in percentage. Assays were repeated a minimum of five times, in triplicate. Enrichment of young human RBCs Whole blood from haemochromatosis patients undergoing phlebotomy therapy was enriched for very young human RBCs as described previously [48] , [49] with minor modifications. After leukocyte removal (Sepacell R-500 filters), the blood was aliquoted in 50-ml tubes and centrifuged (4,000 g /1 h). The top 4 ml of packed blood was collected from each tube and resuspended in serum at 50% haematocrit. Five millilitre aliquots were layered on top of 6 ml of 70% Percoll solution and centrifuged (1,200 g /15 mins) to give a concentrated band of cells enriched for the youngest age group at the interface. The reticulocyte percentage was measured using supravital staining with New Methylene Blue (Sigma) as an estimate of the enrichment level (usually 40% of the obtained RBCs were reticulocytes). Continuous proliferation assay of P. knowlesi H Enriched very young RBCs were added to normocytes to obtain different proportions of young RBCs, represented as percentages of reticulocytes (2%, 4%, 8%, 12% and 16% in average), and plated at 2% haematocrit. P. knowlesi H schizonts were seeded at 1% parasitaemia in these cultures. Every 2 days, the cultures were split back to a parasitaemia of 0.7−1%, and supplemented with appropriate amount of freshly enriched RBCs. Cultures that did not reach a parasitaemia of 1% were split in half. Parasitemia was monitored daily, before and after subculture. Mathematical Model Framework Our mathematical model is similar to previous models that focus on the impact of resource limitation on within-host infection dynamics [24] , [27] , [50] . To describe the dynamics of within-host parasite invasion, three distinct entities are tracked: (i) susceptible RBCs ( S ), (ii) infected RBCs (I) and (iii) free-living merozoites ( M ) released, 24 h after infection for P. knowlesi , and 48 h for P. falciparum and P. vivax . The density of susceptible RBCs in the host increases because of RBC production (b) and decreases because of clearance of senescent cells (with an expected lifespan of 120 days) and invasion by merozoites. The overall rate of invasion, βSM , is assumed to be proportional to the density of merozoites ( M ) and the density of susceptible cells ( S ). The basic set of equations describing this process is: where m is the average number of merozoites released by a bursting cell, μ m is the death rate of merozoites and βS is the parasite invasion rate, which depends on the intrinsic invasion ability β and the density of susceptible cells S (see Table 1 for variable and parameter definitions). Note that growth and development within the cell is modelled as a deterministic process. The effective reproduction number ( R e ) then describes how the proliferation of the parasite depends on host and parasite parameters as follows: Table 1 Parameter definitions and values for within-host mathematical model. Full size table In the absence of immunity, R e in our mathematical model corresponds directly to the laboratory measure of PEMR. By using PEMR, we can directly measure invasion and isolate this from the subsequent growth and development of the parasite within the RBC, consistent with the model structure. The above equations assume that the lifespan of RBCs is exponentially distributed with mean 1/ μ . A more realistic assumption is that the RBC age distribution in a healthy host is approximately uniform, or that most cells live approximately the average lifespan and then are removed by the spleen. To include this assumption, each compartment in the above model is replaced with numerous successive compartments and the system of equations becomes: For each host the rate of release of RBCs from the bone marrow (b) is assumed to be constant and is fixed to ensure that the total RBC density in an uninfected host is 5 million cells per μl. For simplicity, we assume that the age dependence of the intrinsic invasion ability is modelled by a step function and hence for a given age preference there exists an i 0 such that β i = β= constant >0 for all i ≤ i 0 and β i =0 for all i > i 0 . The specific value of β is determined by its relationship to the number of susceptible cells and the basic reproduction number. To simulate the effect of a shifted RBC age distribution within host (see Figs 3c and 5 ), we assumed an increased RBC production in response to haemolytic anaemia, which was modelled by adding an additional mortality (− μ a S i ) term to the right-hand side of each S i equation (that is, the excess cell mortality is experienced by cells of all ages). We assumed that the RBC distribution had reached equilibrium and the increased RBC production was sufficient to compensate for the excess RBC mortality. Hence, at the time of infection, the RBC age distribution of the host will be shifted but the host will have a normal haematocrit. This allows us to separate the effect of anaemia (decreased RBC density) from the effect of shifted RBC age distribution, and therefore likely represents an upper bound for the parasite densities achievable under different levels of RBC skew. A common feature of mathematical models focusing on the impact of resource limitation on within-host malaria infection dynamics is that they overestimate the initial peak parasiteamias [24] , [25] , [50] because they ignore immunity and assume homogenous mixing of merozoites and RBCs. These simplifications allow for the examination of the impact of resource limitations in the absence of confounders. Consistent with this, we assume that a maximum of 5% of all RBCs are susceptible to invasion at any given time, and our model is primarily designed to give insights into relative values. This means that in the model the RBC age classes remain the same, but within each of these age ranges only 5% of all cells are susceptible. If a parasite is restricted to very young cells, the total percentage of cells that are susceptible is then 2%, whereas if a parasite can invade all ages, 5% of all cells are susceptible. 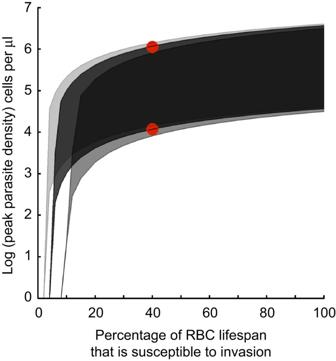Figure 7: Sensitivity analysis for peak parasite densities for an initially healthy host. Each shaded region shows the simulated peak parasite densities for different assumptions about parasite invasion. Moving to the right each shaded region shows how peak parasite density changes as the parasite adapts to be less age restricted. Moving upwards each shaded region shows how peak parasite density changes as the overall percentage of cells that are susceptible (within the susceptible age range) changes from 1 to 100%. Parameter values are chosen so that the middle shaded region corresponds toR0=5, when 40% of the RBC lifespan is susceptible. Note that this implies that the intrinsic invasion abilityβis constant as the parasite age restriction changes but will depend on the maximum overall fraction of susceptible cells. For example, if only 1% of cells within the susceptible age range are susceptible (lower red circle) thenβwill be larger than if 100% of cells within the susceptible age range are susceptible (upper red circle)—in both casesβhas been chosen so thatR0=5. The intrinsic invasion abilityβfor the upper (lower) shaded region are twice (half) the value for the middle shaded region. All other parameter values are the same between regions. Figure 7 shows that our findings hold when no assumption about the upper limit of susceptible cell density is made. Figure 7: Sensitivity analysis for peak parasite densities for an initially healthy host. Each shaded region shows the simulated peak parasite densities for different assumptions about parasite invasion. Moving to the right each shaded region shows how peak parasite density changes as the parasite adapts to be less age restricted. Moving upwards each shaded region shows how peak parasite density changes as the overall percentage of cells that are susceptible (within the susceptible age range) changes from 1 to 100%. Parameter values are chosen so that the middle shaded region corresponds to R 0 =5, when 40% of the RBC lifespan is susceptible. Note that this implies that the intrinsic invasion ability β is constant as the parasite age restriction changes but will depend on the maximum overall fraction of susceptible cells. For example, if only 1% of cells within the susceptible age range are susceptible (lower red circle) then β will be larger than if 100% of cells within the susceptible age range are susceptible (upper red circle)—in both cases β has been chosen so that R 0 =5. The intrinsic invasion ability β for the upper (lower) shaded region are twice (half) the value for the middle shaded region. All other parameter values are the same between regions. Full size image How to cite this article: Lim, C. et al . Expansion of host cellular niche can drive adaptation of a zoonotic malaria parasite to humans. Nat. Commun. 4:1638 doi: 10.1038/ncomms2612 (2013).